High efficiency cell-specific targeting of cytokine activity Systemic toxicity currently prevents exploiting the huge potential of many cytokines for medical applications. Here we present a novel strategy to engineer immunocytokines with very high targeting efficacies. The method lies in the use of mutants of toxic cytokines that markedly reduce their receptor-binding affinities, and that are thus rendered essentially inactive. Upon fusion to nanobodies specifically binding to marker proteins, activity of these cytokines is selectively restored for cell populations expressing this marker. This ‘activity-by-targeting’ concept was validated for type I interferons and leptin. In the case of interferon, activity can be directed to target cells in vitro and to selected cell populations in mice, with up to 1,000-fold increased specific activity. This targeting strategy holds promise to revitalize the clinical potential of many cytokines. Cytokines are small, short-lived proteins that support intercellular communication in numerous key physiological processes. All cytokines function through specific transmembrane receptors and a vast amount of detailed insights into their biological role is at hand. It is clear that several cytokines have considerable clinical potential as antiviral and anticancer agents or to suppress inflammatory and autoimmune conditions [1] . However, the medical use of many cytokines has been severely hampered by their intrinsic, systemic toxicity. The key reason underlying this generalized toxicity is their pleiotropic activity pattern: cytokines often act on most cell types in the body evoking a complex toxicity pattern when administered in high doses. Consequently, the maximum tolerated cytokine doses are far below the optimal therapeutic concentrations. One strategy to circumvent this toxicity problem is the development of so-called immunocytokines: cytokines fused to a binding module such as a scFv-antibody fragment or a nanobody to target them to selected cells [2] . This concept relies on the use of cell-specific, surface-expressed marker proteins that are recognized by the targeting module. The best therapeutic results in preclinical models were obtained for IL-2, IL12, IL15 and TNFα [2] . Although many variations on this theme were developed, the overall, main problem remained that with only a roughly 10-fold increased activity on target compared with untargeted cells, the therapeutic index of these immunocytokines remains still very low. Here we developed a generic approach to increase by several orders of magnitude the targeting efficiency of immunocytokines. We speculated that the rather modest targeting effects are related to the observation that increasing cytokine-binding affinities towards the cell surface in many cases does not increase their potency [3] , [4] , [5] , [6] , [7] . Targeting of immunocytokines is—from a biophysical perspective—based on increasing their binding affinity specifically towards cells expressing a given marker. We envisioned markedly improved targeting efficiencies for immunocytokines by strongly reducing their receptor-binding affinities thus rendering these essentially inactive in the absence of additional binding to a cell marker. Consequently, the activity of such molecules can be restored in a highly selective manner on cells recognized by the targeting module. The proof of this concept was established for type I interferon (IFN) that represents the archetype of a cytokine that may find full clinical potential if it can be properly targeted. Type I IFNs encompass the IFNα subtypes and IFNβ and act through interaction with a ubiquitously expressed receptor composed of IFNAR1 and IFNAR2 subunits. The IFN-receptor complex formation is a two-step reaction that initiates with the formation of an IFN-IFNAR2 binary complex followed by the interaction with IFNAR1 (refs 8 , 9 ). This ternary complex activates a canonical Jak/Stat pathway leading to the expression of IFN-stimulated genes (ISGs). In so doing, IFNs tune a broad range of biological activities directed to non-immune and immune cells and bridge innate and adaptive immune responses [10] . In spite of clear antitumor and antiviral effects in mice, clinical applications of type I IFNs have remained rather disappointing, and whenever possible alternative therapies have been implemented. The main reason for this failure lies in the ubiquitous expression of its receptor, rendering IFN action systemic. The severe side effects experienced by the patients limit the administrable doses and consequently the IFN concentration at the desired site [11] , [12] . Nonetheless, type I IFNs are essential in initiating the immune processes needed to achieve durable tumour rejection and eradication of viral infections [13] , [14] . As for other cytokines, the use of IFNs fused to antibodies resulted in only a 10-fold increased activity towards targeted cells [15] , [16] , and off-target side effects experienced by the patients are expected to remain a major obstacle. The huge potential of targeting IFNs to specific cell types has been recognized early, but so far attempts have failed to achieve sufficient targeting efficiencies [15] , [16] , [17] . Detailed structure, affinity and activity studies have revealed that the binding affinities of IFNs appear optimized to a level that a further increase is not paralleled by enhanced potencies [3] , [18] , [19] . We therefore envisioned obtaining considerably higher targeting efficacies for IFNs with suitably reduced receptor-binding affinities. For this reason, here we employ IFNα2 mutations within the binding site for the high-affinity subunit IFNAR2, which reduce their potency by a factor of 10–200 compared with WT IFNα2 (ref. 20 ). For specific targeting, these mutants are fused to nanobodies (Nbs) directed against a cell surface antigen. Nbs combine the assets of conventional antibodies with advantageous properties such as small size, high stability and easy manufacturing [21] . We show here that such engineered IFNs recover almost maximally their bioactivities uniquely on the targeted cells, exhibiting up to 3 log targeting efficiency, both in vitro and in vivo when delivered in mice. Decreasing IFN-receptor affinity enhances targeting In order to establish the proof of the ‘activity-by-targeting’ concept for type I IFNs, we first fused a nanobody (Nb) 4.11 (ref. 22 ) directed against the murine leptin receptor (mLepR) to either WT human IFNα2 or the R149A mutant. This mutation reduces the affinity of IFN to its receptor by a factor 200 by increasing its dissociation rate constant of the interaction with IFNAR2, keeping the IFN-IFNAR2 on-rate and the IFN-IFNAR1 affinity intact [20] . The overall architecture of the fusion proteins is depicted in Fig. 1a . These proteins were produced in insect cells and purified to homogeneity ( Supplementary Fig. S1 ). The rate constants and binding affinities of these fusion proteins towards the extracellular domain of IFNAR2 were confirmed by real-time solid phase detection ( Supplementary Fig. S2 ). Both immunocytokines were assayed, together with the parental IFNα2 and IFNα2-R149A, on HL116 cells, a clone containing an IFN-inducible firefly luciferase reporter gene [23] , and on the HL116-mLR10 clone that stably expresses the mLepR ( Fig. 1b ). The IFNα2-R149A mutant is approximately 200-fold less active on both HL116 and HL116-mLR10 cell lines, which was expected since the specific activity of IFNα is directly proportional to its affinity for IFNAR1 and IFNAR2 (ref. 18 ). We also found that the fusion with the Nb reduces the potency of IFN by a factor 10. As a result, the specific activity of the Nb4.11-IFNα2-R149A fusion protein represents ~0.05% of the original IFNα2 activity on HL116 cells. Strikingly, its activity is largely recovered when assayed on HL116-mLR10 cells. The resulting 800-fold targeting efficiency of the Nb4.11-IFNα2-R149A immunocytokine is sufficiently large to predict therapeutic dosing inducing a maximal effect (90%) in cells expressing the Nb target antigen and only a marginal effect (1%) on non-targeted cells. The targeting efficiency is directly linked to the impact of the R149A mutation since two other mutations, L153A and M148A, which have an intermediate effect on the IFN-IFNAR2 interaction ( Supplementary Table S1 ), display proportionally reduced targeting efficiencies ( Fig. 1c ). These results corroborate that indeed the drastically reduced intrinsic potency of the mutant immunocytokine is key for efficient targeting. 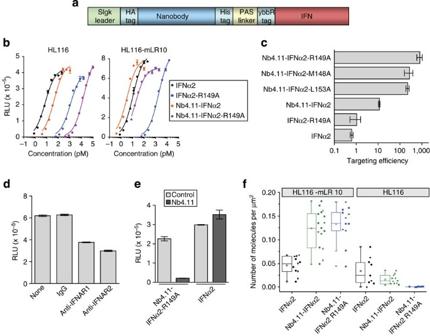Figure 1: High efficiency targeting of IFN activity on cells expressing the mLepR. (a) Schematic representation of the Nb-IFN fusion proteins. (b) Induction of luciferase activity in HL116 cells (left panel) or in HL116-mLR10 cells which express the mLepR (right panel) by IFNα2 (black symbols), IFNα2-R149A (blue symbols) or by these IFNs fused to the Nb4.11 specific for the mLepR (orange and purple symbols). Luciferase activity is expressed as relative luminescence units (RLU). Each point represents the mean of three replicates and s.e.m. (c) The targeting efficiency of the indicated IFN or Nb4.11-IFN fusion proteins is shown as the ratio of the EC50values obtained on HL116 and HL116-mLR10 cells. Mean of three to six independent assays, error bars are s.e.m. (d) Effect of 5 μg ml−1of neutralizing antibodies against IFNAR1 and IFNAR2 or control IgG on the luciferase activity induced by 220 pM of Nb4.11-IFNα2-R149A on HL116-mLR10 cells. Each value represents the mean of three replicates and s.e.m. (e) Effect of 170 nM of unconjugated 4.11 Nb on the luciferase activity induced by 650 pM of Nb4.11-IFNα2-R149A or 10 pM of IFNα2 on HL116-mLR10 cells. Each value represents the mean of three replicates and s.e.m. (f) Binding of fluorescent Nb4.11-IFNα2 and Nb4.11-IFNα2-R149A to HL116-mLR10 cells and to HL116 cells quantified by single-molecule imaging. For comparison, binding of IFNα2 to both cell lines is shown. The box represents the 25 and 75 percentile, the line in the middle of the box the 50 percentile (median), the square the mean, the whiskers 1.5 of the interquartile range and x the outliers of the data. Figure 1: High efficiency targeting of IFN activity on cells expressing the mLepR. ( a ) Schematic representation of the Nb-IFN fusion proteins. ( b ) Induction of luciferase activity in HL116 cells (left panel) or in HL116-mLR10 cells which express the mLepR (right panel) by IFNα2 (black symbols), IFNα2-R149A (blue symbols) or by these IFNs fused to the Nb4.11 specific for the mLepR (orange and purple symbols). Luciferase activity is expressed as relative luminescence units (RLU). Each point represents the mean of three replicates and s.e.m. ( c ) The targeting efficiency of the indicated IFN or Nb4.11-IFN fusion proteins is shown as the ratio of the EC 50 values obtained on HL116 and HL116-mLR10 cells. Mean of three to six independent assays, error bars are s.e.m. ( d ) Effect of 5 μg ml −1 of neutralizing antibodies against IFNAR1 and IFNAR2 or control IgG on the luciferase activity induced by 220 pM of Nb4.11-IFNα2-R149A on HL116-mLR10 cells. Each value represents the mean of three replicates and s.e.m. ( e ) Effect of 170 nM of unconjugated 4.11 Nb on the luciferase activity induced by 650 pM of Nb4.11-IFNα2-R149A or 10 pM of IFNα2 on HL116-mLR10 cells. Each value represents the mean of three replicates and s.e.m. ( f ) Binding of fluorescent Nb4.11-IFNα2 and Nb4.11-IFNα2-R149A to HL116-mLR10 cells and to HL116 cells quantified by single-molecule imaging. For comparison, binding of IFNα2 to both cell lines is shown. The box represents the 25 and 75 percentile, the line in the middle of the box the 50 percentile (median), the square the mean, the whiskers 1.5 of the interquartile range and x the outliers of the data. Full size image Activity of targeted IFN depends on both IFNAR and Nb target Neutralizing antibodies against IFNAR1 and IFNAR2, as well as the unconjugated 4.11 Nb, inhibit the targeting of the Nb4.11-IFNα2-R149A construct on HL116-mLR10 cells ( Fig. 1d,e ). Single-molecule fluorescence imaging with Nb–IFN fusion proteins site-specifically labelled via their ybbR-tag ( Supplementary Fig. S3 ) revealed similar binding of Nb4.11-IFNα2-R149A and Nb4.11-IFNα2 to HL116-mLR10 cells ( Fig. 1f ), suggesting that binding was dominated by the Nb-mLepR interaction. Indeed, strong and highly stable binding of Nb4.11-IFNα2-R149A to the mLepR was confirmed for HL116-mLR10 cells even after blocking IFNAR binding sites with IFN ( Supplementary Fig. S4 ). In contrast, markedly less binding of Nb4.11-IFNα2-R149A compared with Nb4.11-IFNα2 was observed for HL116 cells ( Fig. 1f ). HL116-mLR10 cells (which express an IFN-inducible firefly luciferase gene) were co-cultured at confluency in a 1:1 ratio with a non-targeted cell line expressing an IFN-inducible Renilla luciferase gene in the presence of 220 pM of the Nb4.11-IFNα2-R149A. At this IFN concentration, a maximal response on targeted cells and a marginal effect on non-targeted cells are expected to be induced (see Fig. 1b ). Accordingly, only firefly luciferase activity can be detected ( Fig. 2a ). This indicates that the targeted IFN acts exclusively on mLepR-expressing cells and does not exert any activity in trans, that is, towards neighbour cells that do not express the target. Finally, we also evaluated whether topological constraints may determine the efficiency of this targeting effect. This is not the case as shown in Fig. 2b since Nbs that bind different extracellular domains of the mLepR [22] evoke the same effect. 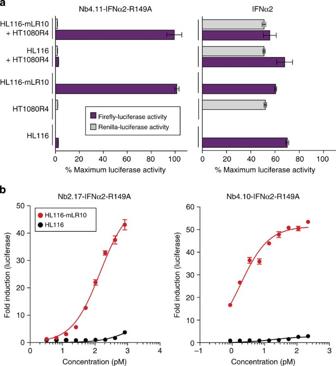Figure 2: The targeting effect is exerted only incisand is not affected by the location of the Nb epitope. (a) Cells expressing an IFN-inducible firefly luciferase (HL116) or HL116-mLR10 cells were co-cultured at a 1:1 ratio with an HT1080 cell clone expressing an IFN-inducible renilla luciferase (HT1080R4). The two co-cultures and single-cell type control cultures were treated with 220 pM Nb4.11-IFNα2-R149A (left panel), a dose that induces a maximal response in cells carrying the mLepR and a minimal response on cells devoid of the Nb target, or 7 pM IFNα2 (right panel). After 6 h, the induced renilla and firefly luciferase activities were quantified. Results are expressed as the percentage of the maximum activity induced by an excess concentration of IFN (2.2 nM Nb4.11-IFNα2-R149A or 3.4 nM IFNα2). Each histogram represents the mean of three replicates and s.e.m. The experiment shown is representative for three. (b) Induction of luciferase activity in HL116 (black symbols) or in HL116-mLR10 (red symbols) cells by IFNα2-R149A fused either to the Nb2.17 (left panel) or to the Nb4.10 (right panel) that bind different extracellular domains of the mLepR. Results are expressed as fold induction (Nb-IFN fusion proteins treated cells versus non treated cells). Each value represents the mean of three replicates and s.e.m. Figure 2: The targeting effect is exerted only in cis and is not affected by the location of the Nb epitope. ( a ) Cells expressing an IFN-inducible firefly luciferase (HL116) or HL116-mLR10 cells were co-cultured at a 1:1 ratio with an HT1080 cell clone expressing an IFN-inducible renilla luciferase (HT1080R4). The two co-cultures and single-cell type control cultures were treated with 220 pM Nb4.11-IFNα2-R149A (left panel), a dose that induces a maximal response in cells carrying the mLepR and a minimal response on cells devoid of the Nb target, or 7 pM IFNα2 (right panel). After 6 h, the induced renilla and firefly luciferase activities were quantified. Results are expressed as the percentage of the maximum activity induced by an excess concentration of IFN (2.2 nM Nb4.11-IFNα2-R149A or 3.4 nM IFNα2). Each histogram represents the mean of three replicates and s.e.m. The experiment shown is representative for three. ( b ) Induction of luciferase activity in HL116 (black symbols) or in HL116-mLR10 (red symbols) cells by IFNα2-R149A fused either to the Nb2.17 (left panel) or to the Nb4.10 (right panel) that bind different extracellular domains of the mLepR. Results are expressed as fold induction (Nb-IFN fusion proteins treated cells versus non treated cells). Each value represents the mean of three replicates and s.e.m. Full size image Antiviral activity of mutant IFN on targeted cells In order to confirm efficient IFN targeting on the level of cellular responses, we probed for antiviral protection by Nb-IFN, the hallmark of IFN function. 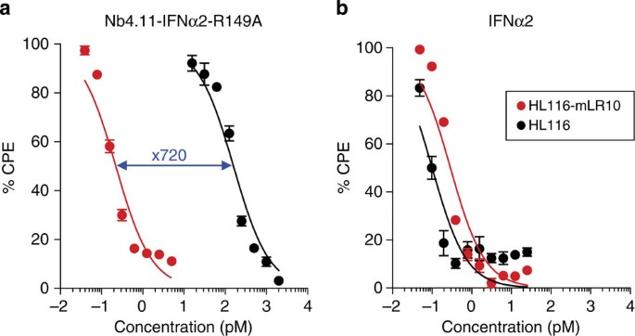Figure 3: The Nb4.11-IFNα2-R149A exerts an antiviral effect specifically on mLepR-expressing cells. Antiviral activity of Nb4.11-IFNα2-R149A (a) and IFNα2 (b) for the inhibition of the cytopathic effect of the EMC virus on HL116 cells (black symbols) or HL116-mLR10 cells (red symbols). Each value represents the mean of six replicates and s.e.m. Figure 3 shows that a Nb-mutant IFN chimera is able to establish an antiviral state in targeted cells. Indeed, the Nb4.11-IFNα2-R149A construct is 720-fold more potent in inhibiting the replication of encephalomyocarditis virus in targeted cells compared with cells not expressing the Nb target, whereas both cell lines show similar responsiveness to WT IFNα2. Since antiviral activity is representative of an integrated IFN response, which needs the coordinated action and the stability of expression of several IFN-sensitive genes (ISGs), this result corroborates that the IFN activity delivered on targeted cells by the mutant immunocytokine has the potential to induce full IFN responses. Figure 3: The Nb4.11-IFNα2-R149A exerts an antiviral effect specifically on mLepR-expressing cells. Antiviral activity of Nb4.11-IFNα2-R149A ( a ) and IFNα2 ( b ) for the inhibition of the cytopathic effect of the EMC virus on HL116 cells (black symbols) or HL116-mLR10 cells (red symbols). Each value represents the mean of six replicates and s.e.m. Full size image Targeting of other cytokine activities Having in detail verified the concept of ‘activity-by-targeting’ for IFNs in vitro and in vivo , we aimed to demonstrate generic application. In Fig. 4 , we apply the same principle to leptin. Leptin activates a homomeric receptor complex by bridging a cytokine receptor homology domain (CRH2) and an immunoglobulin-like domain (Ig) of two receptor chains. The murine leptin mutants L86S or L86N, with respectively moderately and strongly reduced affinity for CRH2 (ref. 24 ) were fused to a Nb targeting human tumour necrosis factor receptor 1 (TNFR1) (Nb96) by means of a GGS linker sequence ( Fig. 4a ). As shown in Fig. 4b , Ba/F3 cells that stably express the mouse leptin receptor and human TNFR1 (lacking its cytosolic domain to abrogate downstream signalling) strongly respond to Leptin-L86S-Nb96, whereas only a very limited effect can be observed on BaF/3 cells only expressing the leptin receptor. Similarly, a profound ‘activity-by-targeting’ effect was observed for selected mutant interleukin-1/Nb and tumour necrosis factor alpha (TNFα)/Nb immunocytokines (will be published elsewhere). 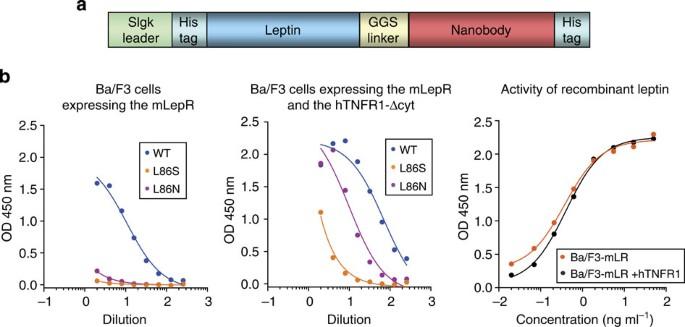Figure 4: Targeting of leptin activity. (a) Schematic representation of the Nb-leptin fusion proteins. (b) Cell proliferation assays: Ba/F3 cells expressing the mLepR (left panel) and Ba/F3 cells expressing the mLepR and the hTNFR1-Δcyt (middle panel) were treated with two fold dilution series using conditioned medium from HEK293T cells expressing the fusion proteins of the anti-hTNFR1 nanobody with wild-type leptin (blue) or leptin mutant L86S (orange) or leptin mutant L86N (purple). Proliferation was monitored after 4 days by the addition of XTT that is converted by living cells to a water soluble formazan salt and measured at 450 nm. Right panel: activity of recombinant leptin on Ba/F3 cells expressing the mLepR and the hTNFR1-Δcyt. The experiment shown is representative for four. Figure 4: Targeting of leptin activity. ( a ) Schematic representation of the Nb-leptin fusion proteins. ( b ) Cell proliferation assays: Ba/F3 cells expressing the mLepR (left panel) and Ba/F3 cells expressing the mLepR and the hTNFR1-Δcyt (middle panel) were treated with two fold dilution series using conditioned medium from HEK293T cells expressing the fusion proteins of the anti-hTNFR1 nanobody with wild-type leptin (blue) or leptin mutant L86S (orange) or leptin mutant L86N (purple). Proliferation was monitored after 4 days by the addition of XTT that is converted by living cells to a water soluble formazan salt and measured at 450 nm. Right panel: activity of recombinant leptin on Ba/F3 cells expressing the mLepR and the hTNFR1-Δcyt. The experiment shown is representative for four. Full size image Targeting IFN activity on mouse primary cells We next studied the effect of Nb-targeted IFN on primary mouse cells. For this purpose, we changed both the Nb and the IFN since the mLepR is ubiquitously expressed and since human IFNα2 is not active on mouse cells due to too low affinities for both murine IFNAR1 and IFNAR2 (refs 25 , 26 ). A single Q124R mutation in human IFNα2 has been shown to render it active on mouse cells but at a 100-fold lower level when compared with murine IFN [27] . This low specific activity (7,4.10 5 units mg −1 ) is likely to be the consequence of an increased affinity of the human IFNα2 mutant for the murine IFNAR1 chain and a suboptimal interaction with IFNAR2 (ref. 18 ). Such a resemblance with the binding characteristics of IFNα2-R149A on human cells prompted us to assay whether the IFNα2-Q124R mutant would exhibit efficient Nb-dependent targeting towards mouse cells. As a Nb, we chose Nb122 that has been raised against murine programme cell death 1 ligand 2 (PD-L2). The architecture of the resulting immunocytokine is analogous to that depicted in Fig. 1a . PD-L2 is a cell surface protein expressed in a subset of hematopoietic cells and especially in 20% of the B-cell population residing in the mouse peritoneal cavity [28] , [29] ( Supplementary Fig. S5 ). Cells from one mouse peritoneal cavity were collected and treated ex vivo with either 10,000 units ml −1 of murine type I IFN as a positive control, 1 nM of the human IFNα2-Q124R fused to Nb122 or to a Nb targeting green fluorescent protein (GFP) as a negative control. Cells were then stained for PD-L2 expression and for STAT1-pY701 as a marker for the IFN response and analysed by fluorescence-activated cell sorting (FACS). 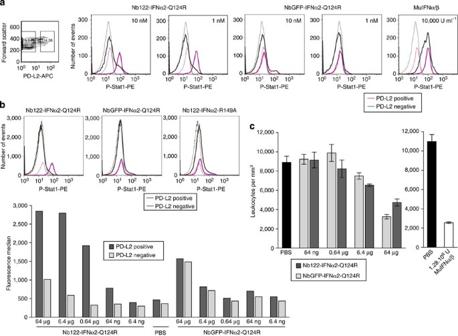Figure 5:Ex vivoandin vivotargeting of IFN activity on mouse tissues. (a) Cells from the peritoneal cavity of C57Bl/6 mice were collected and treatedex vivofor 30 min. with 10,000 units ml−1of natural murine IFNα/β, 1 or 10 nM of Nb122-IFNα2-Q124R or the control NbGFP-IFNα2-Q124R. Left panel: selection of the PD-L2-negative and -positive cell populations. Y701 STAT1 phosphorylation was analysed by FACS in both the PD-L2-negative and PD-L2-positive cell populations. Pink histograms represent P-STAT1 events in the PD-L2-positive cell population, grey histograms for the PD-L2-negative cell population. Plain lines are for cells treated with the indicated IFN, dotted lines are for untreated cells. The X-axis on the left panel and on the histograms represents fluorescence intensity. (b) Similar experiment as in (a), but mice were injected intravenously with the indicated Nb-IFN fusion proteins. PD-L2-negative and -positive cell populations from mice peritoneal cavities were analysed after 45 min by FACS for P-STAT1. The three horizontal upper histograms show FACS data for mice injected with 0.64 μg of the Nb122-IFNα2-Q124R, the control NbGFP-IFNα2-Q124R or the Nb122-IFNα2-R149A construct, which is totally non-active on mouse cells. Data from mice injected with PBS are shown as dotted lines. The X-axis on the histograms represents fluorescence intensity. The bottom panel shows the median of P-STAT1 fluorescence measured in PD-L2-negative (light grey) and -positive (dark grey) cell populations (89,000 to 104,000 and 14,000 to 25,000 events analysed, respectively) of mice injected with the indicated amount of Nb122-IFNα2-Q124R or NbGFP-IFNα2-Q124R. The Y-axis (fluorescence median) represents the median of the overall fluorescence signal obtained when cells from mouse peritoneal cavity were stained with PE-labelled anti-STAT1(pY701) and analysed by flow cytometry. (c) Right panel: leukocyte count in peripheral blood of mice 4 h after i.v. injection of the indicated amount of Nb122-IFNα2-Q124R or NbGFP-IFNα2-Q124R. Left panel: in a separate experiment, the effect of natural murine IFNα/β was evaluated. Mean values and s.e.m. of counts from three to nine mice in each group. Figure 5a shows that Nb122-IFNα2-Q124R induces STAT1 phosphorylation only in the PD-L2-positive cell population, whereas untargeted murine IFN acts on both PD-L2-positive and -negative cells. A similar result was obtained on mouse splenocytes where the PD-L2-positive cell population represents less than 1% of the total cells ( Supplementary Fig. S6 ). These results confirmed that, as predicted, the low receptor affinity of human IFNα2-Q124R makes it suitable for activity-by-targeting on mouse cells. Figure 5: Ex vivo and in vivo targeting of IFN activity on mouse tissues. ( a ) Cells from the peritoneal cavity of C57Bl/6 mice were collected and treated ex vivo for 30 min. with 10,000 units ml −1 of natural murine IFNα/β, 1 or 10 nM of Nb122-IFNα2-Q124R or the control NbGFP-IFNα2-Q124R. Left panel: selection of the PD-L2-negative and -positive cell populations. Y701 STAT1 phosphorylation was analysed by FACS in both the PD-L2-negative and PD-L2-positive cell populations. Pink histograms represent P-STAT1 events in the PD-L2-positive cell population, grey histograms for the PD-L2-negative cell population. Plain lines are for cells treated with the indicated IFN, dotted lines are for untreated cells. The X-axis on the left panel and on the histograms represents fluorescence intensity. ( b ) Similar experiment as in ( a ), but mice were injected intravenously with the indicated Nb-IFN fusion proteins. PD-L2-negative and -positive cell populations from mice peritoneal cavities were analysed after 45 min by FACS for P-STAT1. The three horizontal upper histograms show FACS data for mice injected with 0.64 μg of the Nb122-IFNα2-Q124R, the control NbGFP-IFNα2-Q124R or the Nb122-IFNα2-R149A construct, which is totally non-active on mouse cells. Data from mice injected with PBS are shown as dotted lines. The X-axis on the histograms represents fluorescence intensity. The bottom panel shows the median of P-STAT1 fluorescence measured in PD-L2-negative (light grey) and -positive (dark grey) cell populations (89,000 to 104,000 and 14,000 to 25,000 events analysed, respectively) of mice injected with the indicated amount of Nb122-IFNα2-Q124R or NbGFP-IFNα2-Q124R. The Y-axis (fluorescence median) represents the median of the overall fluorescence signal obtained when cells from mouse peritoneal cavity were stained with PE-labelled anti-STAT1(pY701) and analysed by flow cytometry. ( c ) Right panel: leukocyte count in peripheral blood of mice 4 h after i.v. injection of the indicated amount of Nb122-IFNα2-Q124R or NbGFP-IFNα2-Q124R. Left panel: in a separate experiment, the effect of natural murine IFNα/β was evaluated. Mean values and s.e.m. of counts from three to nine mice in each group. Full size image Targeting IFN activity in vivo on PD-L2-expressing cells We next evaluated whether IFN activity can be targeted in vivo in mice. For this purpose, mice received an intravenous injection with either IFNα2-Q124R linked to the anti PD-L2 or GFP Nb, murine type I IFN or a chimera consisting of Nb122 fused to IFNα2-R149A, which is totally inactive on mouse cells. Peritoneal cells ( Fig. 5b ) and splenocytes ( Supplementary Fig.S7 ) were collected 45 min after the injection and analysed by FACS for activation of STAT1 in PD-L2-positive and -negative cell populations. Strongly enhanced STAT1 phosphorylation in PD-L2-positive compared with PD-L2-negative cells was observed for Nb122-IFNα2-Q124R, but not for NbGFP-IFNα2-Q124R. Thus, ~75% of the maximum STAT1 activation was obtained by 0.64 μg Nb122-IFNα2-Q124R in PD-L2-positive cells, while no activation was detectable in PD-L2-negative cells at this dose. This analysis clearly demonstrated that Nb122-IFNα2-Q124R can be used in vivo to selectively deliver IFN activity on PD-L2-expressing cells. IFN-induced leukopenia—that is, the loss of leukocytes—is one of the side effects encountered by the patients during IFN therapy [12] and is also evident in IFN-treated mice [30] . Figure 5c shows peripheral blood leukocyte counts in mice injected intravenously with the indicated dose of Nb122-IFNα2-Q124R and NbGFP-IFNα2-Q124R. Data indicate that the Nb-IFNα2-Q124R doses that induce leukopenia match the doses inducing IFN activity on non-targeted cells. Indeed, at a dose of 0.64 μg Nb122-IFNα2-Q124R suitable for inducing a strong, targeted activity ( Fig. 5b ), no effect on leukocyte counts was observed. This supports the possibility of clinical applications of a targeted IFN without inducing off-target side effects. Antibody-mediated accumulation of drugs within specific tissues or tumours has emerged as an effective strategy for reducing toxic side effects. For the delivery of cytokines, however, this approach has yielded rather disappointing targeting efficiencies. Traditional immunocytokines have been generated by fusing antibody fragments such as scFv or Nb to WT cytokines. This concept was applied to IFN by several groups who showed that the IFN fusion retained both antigen binding and bioactivities. When studied in vivo , the immuno-IFN was found to be enriched at the targeted site [15] , [16] , [17] . Yet, only 10-fold higher potency on cells expressing the target compared with untargeted cells has been achieved. A low targeting efficiency is also found for the IL-2 immunocytokine under clinical development, which achieves therapeutic effects comparable to the ones observed by the cytokine alone at only a 20-fold lower-administered dose [2] . These rather modest targeting effects relate to the fact that increasing the binding affinity of cytokines towards its receptor does not necessarily augment its potency as previously demonstrated by protein engineering for several cytokines [3] , [4] , [5] , [6] , [7] , [19] . Non-equilibrium binding due to endocytosis and endosomal trafficking of signalling complexes has been suggested to be responsible for such ‘saturation’ behaviour [4] . Cell type-specific targeting of cytokines by fusion to a protein module binding to a surface marker is mainly based on stabilizing the interaction with the cell surface receptor by avidity, that is, by specifically increased affinity towards target cells [31] . For cytokines with saturated binding affinities, however, this targeting strategy is largely in vain as the increase in binding does not pay off in increased potency on target cells. Using IFN as a paradigm for medically relevant cytokine activity, we have here systematically devised and tested a generic strategy to overcome this limitation by using cytokine mutants with considerably reduced affinities and potencies. We demonstrated that such a mutated IFN immunocytokine is up to almost 1,000-fold more potent on cells expressing a selected target at their surface and show that our targeting strategy delivers activity only to the selected cells when injected intravenously in mice. Such an exceptionally high in vivo targeting efficiency is due to an increased cell surface binding achieved by Nb-mediated interaction that compensates the reduced IFN activity specifically on cells expressing the Nb target protein. As a result, the immunocytokine is virtually inactive while ‘en route’ and is activated only upon binding to the desired target. This property is important for the clinical use of immunocytokines in general and is particularly appropriate in the case of IFN, which acts in the pM concentration range on all cell types [2] , [17] , [32] , [33] . Importantly, we found that the targeting effect is exerted only in cis and not in trans on nearby cells and appears robust with respect to the nature of the target protein and the location of the Nb epitope. Given the need to maximally reduce toxic side effects due to systemic IFN activity, efficient targeting of IFN may find clinical application in various ways. Depending on the Nb chosen, targeting of tumour cells, virally infected cells or particular immune effector or regulatory cells can all be envisioned. In addition, combination therapies may very well ameliorate the clinical outcome of dendritic cell vaccination, adoptive T-cell therapy, as well as various types of radio-, chemo- and immuno-therapies since the efficacy of these clinical practices often depends on endogenous IFN [13] , [34] , [35] . Finally, since binding affinities of many natural cytokines appear to have evolved to a maximum potency, increasing their targeting specificity by using mutants with reduced binding affinity is likely to prove valuable as well. The only additional prerequisite compared with classical immunocytokine strategies is the availability of mutants with sufficiently reduced receptor-binding affinity, which may prove somewhat more complicated in the case of promiscuous ligands engaging multiple receptors. Strikingly, the same concept was without any further optimization readily transferred to leptin, a functionally unrelated cytokine. Moreover, we already could extend this ‘activity-by-targeting’ effect to interleukin-1 and TNFα, two structurally unrelated cytokines, further supporting the generic applicability of this strategy. Construction of the Nb-IFNα2 fusions The IFNα2 and the mutants L153A, M148A and R149A were cloned in the pT3T7 vector (Stratagene) in fusion with the ybbR-tag sequence at their N-term [36] . The ybbR-IFN sequences were amplified by a PCR Expand High Fidelity PCR system (Roche Diagnostics) and the following primers: Forward: 5′-GGGGGGTCCGGACCATCACCATCACCATCACCATCACCATCACCCTGCTTCTCCC GCCTCCCCAGCATCACCTGCCAGCCCAGCAAGTGATAGCCTGGAATTTATTGC-3′, Reverse: 5′-CGTCTAGATCATTCCTTACTTCTTAAAC-3′ in order to introduce a His tag sequence and a repeat of a sequence encoding five Pro-Ala-Ser residues at the 5′-end of the ybbR-IFNs. The PCR products were digested with Bsp EI and Xba I and cloned at the 3′-end of the sequences encoding nanobody (Nb) against the murine leptin receptor (mLepR) 4.10, 4.11 or 2.17, themselves cloned in fusion with the SIgK leader peptide sequence and the HA tag sequence into the pMET7 vector [22] . In order to construct pMET7 vector encoding Nb-PD-L2-IFN or NbGFP-IFN fusions, the Nb-encoding sequence of Nb-mLepR-IFN constructs was swapped with the sequences encoding Nb-PD-L2 or Nb-GFP obtained by PCR amplification from the plasmid pHEN6c-4PDII-122 or pcDNA3-GFP-VHH, respectively. The mutation Q124R was introduced into the IFNα2 sequence by site-directed mutagenesis using the QuikChange II-E Site-Directed Mutagenesis Kit (Agilent Technologies). All Nbs were generated at the VIB Protein Service Facility as described previously [22] . Construction and production of the mLeptin-Nb fusions Plasmid construct for the production of the fusion proteins consisting of mouse leptin and a nanobody against human tumour necrosis factor receptor 1 (TNFR1) (nb96; gift Dr C. Libert) were made in the pMet7 expression vector. Mouse leptin (wt or mutants) were fused to the N-terminus of nb96 by means of a (GGS)n ( n =18 or 20) linker. The signal peptide for cellular secretion was from Ig kappa V-region. Fusion constructs were made with leptin mutants L86S and L86N shown to have moderate and strong reduced affinity for the leptin receptor, respectively [24] . Hek293T cells (ATCC CRL-11268) were transiently transfected using lipofectamine (Invitrogen), and the supernatant was collected 4 days later, filtered and used for cell proliferation assays. Generation of cell lines stably expressing TNFR1 Ba/F3 cells (DSMZ ACC 300) stably expressing the mouse leptin receptor (mLepR) were selected for growth in the presence of leptin. These cells were additionally transfected with the human TNFR1 (p55) lacking its intracellular domain (hTNFR1-Δcyt). A pool of TNFR1-positive cells was obtained by cotransfection of a plasmid conferring resistance to puromycin followed by FACS after staining with a mAB specific for the human TNFR1(R&D Systems; MAB225). Nb-IFN fusions production and purification Small scale Nb-IFN productions were obtained by harvesting conditioned medium of Hek293T cells transiently transfected by lipofectamine (Invitrogen) with the pMET7-Nb-vectors. Nb-IFN fusions were purified using the HisPur Ni-NTA purification kit (Thermo scientific). For large scale production in insect cells, the sequences encoding the Nb-IFN fusions were subcloned into the pBAC-3 vector (Novagen) suitable for protein secretion into the medium. Baculovirus were generated by coinfection with linearized viral DNA (BD Biosciences) into Sf9 cells. Protein expression was carried out in Hi5 cells infected at a multiplicity of infection of ~10. Cell supernatants were collected 3-4 days post infection, dialyzed against 20 mM TRIS pH 8, 200 mM NaCl and purified by immobilized metal ion chromatography (IMAC) on a HisTrap Sepharose resin loaded with Zn(II) ions using imidazole for elution [37] . For biophysical studies, proteins were further purified by size-exclusion chromatography on a Superdex 200 column. Nb-IFN fusion proteins were labelled with DY647 via the ybbR-tag by enzymatic phosphopantetheinyl transfer (PPT) followed by size-exclusion chromatography as described earlier [38] . For ex vivo and in vivo targeting experiments, proteins were incubated with 10 units ml −1 benzonase for 30 min at room temperature in order to deplete nucleic acid contaminations, and subsequently purified by IMAC as described above. Imidazole was removed by dialysis in 20 mM HEPES pH 8, 100 mM NaCl. Concentration of large scale productions was determined by measuring the absorbance at 280 nm. The concentration of small scale productions was determined by a sandwich ELISA assay using a mouse anti-HIS and a rat anti-HA antibody (Sigma Aldrich and Roche diagnostic, respectively) and a biotin-anti mouse IgG (Jackson) plus streptavidin HRP (BD Biosciences). A construct with a concentration determined by absorbance at 280 nm was used as standard. The biological activities of all products were assessed by functional assays using either the luciferase reporter cell lines HL116 (human) or LL171 (mouse) against human IFNα2c (from Dr G. Adolf, Ernst Boehringer Institute, Vienna, Austria) or the WHO International mouse IFNα standard Ga02-901-511 (bei resources) as described previously [23] . IFN binding assays The interaction of Nb-IFN fusion proteins with the extracellular domain of IFNAR2 (IFNAR2-EC) was probed in vitro by real-time surface-sensitive detection using simultaneous total internal reflection fluorescence spectroscopy and reflectance interference (TIRFS-RIF) detection using a setup described before [39] , [40] . IFNAR2-EC fused to an ybbR-tag was immobilized onto a Coenzyme A-functionalized surface via enzymatic phosphopantetheinyl transfer as described previously [38] . Subsequently, binding of fluorescence-labelled Nb-IFN fusion proteins injected at 100 nM concentration was monitored by TIRFS. Binding of fluorescent Nb-IFN to the cell surface was probed on the single-molecule level by total internal reflection fluorescence microscopy. Measurements were carried out in an Olympus IX 71 microscope equipped with a total internal reflection condenser, a 642 nm diode laser (140 mW output, Omicron) and an EMCCD camera (iXon DU897D, 512 × 512 pixel from Andor Technology) [41] . For binding experiments, cells were grown on cover slides coated with poly- L -lysine-graft-polyethylene glycol copolymer functionalized with RGD peptide for minimizing non-specific binding. Proteins labelled with Dy647 were incubated at typical concentrations of 2 nM and imaged in the presence of an oxygen scavenger cocktail. Leptin-induced proliferation assay Ba/F3 cells expressing both the mLepR and the hTNFR1-Δcyt, or mLepR alone were plated at 5,000 to 10,000 cells per well in 96-well plates. Serial dilutions of leptin or fusion proteins were added, and 4 days later cell proliferation was assessed by using the XTT method (Roche Diagnostics; XTT cell proliferation kit II). IFN-induced luciferase assays The HL116 clone [23] is derived from the human HT1080 cell line (ATCC CCL-121). It contains the firefly luciferase gene controlled by the IFN-inducible 6-16 promoter. HL116 cells were co-transfected with an expression vector encoding the short isoform of the mLepR (pMET7 mLRsh-FLAG) [42] and pSV2neo using the standard calcium phosphate procedure. Stable transfected clones were isolated in G418-containing medium. The clone 10 was selected after analysis of the surface expression level of the murine leptin receptor by FACS, using 3 μg ml −1 of the biotinylated antimouse leptin receptor antibody (polyclonal goat IgG BAF497 from R&D) and streptavidin-APC (BD biosciences). HT1080 cells were co-transfected with p6-16-RL, a plasmid encoding the Renilla luciferase (from pRL-null, Promega) controlled by the IFN-inducible 6-16 promoter from p1.8gpt-5 (ref. 43 ), pBB3 (ref. 44 ) and sonicated salmon sperm DNA (Sigma Aldrich). Stable transfected clones were isolated in HAT-containing medium. The clone 4 (HT1080R4) was selected for a high level of Renilla luciferase activity induction upon IFN stimulation. Luciferase activities were determined on a Berthold centro LB960 luminometer using either the Firefly Luciferase Assay System or the Dual-Luciferase Reporter Assay System (Promega) after 6 h IFN stimulation. EC 50 was calculated by non-linear regression of the dose–response curves using Prism software (GraphPad). The inhibition of the IFN-induced IFN activity was obtained using the anti-IFNAR1 mAb 64G12 (a generous gift of Dr. P. Eid, INSERM, Villejuif, France), the anti-IFNAR2 mAb MMHAR2 (PBL Interferon Source) or the anti-mLepR Nb 4.11 (ref. 22 ). All cells were cultured in DMEM medium supplemented with 10% fetal calf serum. IFN antiviral assay HL116 and HL116-mLR10 cells were treated overnight with different IFN or Nb-IFN concentrations. The medium was then replaced with encephalomyocarditis virus at a multiplicity of infection of 0.01, and the cytopathic effect was scored as a function of IFN concentration when the control cultures showed 100% destruction as previously described [23] . Phospho STAT1 assay in mice C57Bl/6 mice were obtained from Harlan. All experiments were carried out following the protocol CEEA-LR-11056 approved by the Animal Care and Use Committee Languedoc-Roussillon. Seven- to nine-week-old female mice were injected intravenously through the retro-orbital vein with the indicated amount of Nb-IFN or natural mouse IFNα/β (a generous gift of I. Gresser, INSERM, Paris, France). Forty-five minutes later, mice were killed and single-cell suspensions were prepared from spleens and peritoneal washout fluids as described [29] . Erythrocytes were depleted using red blood cell lysis buffer (Lonza). Isolated cells were labelled with the BD Phosflow PE mouse anti-STAT1 (pY701) together with the APC-labelled rat anti mouse CD273 (programme cell death 1 ligand 2 or PD-L2) according to BD Biosciences instructions. Alternatively, for ex vivo studies, splenocytes or peritoneal cells were treated for 30 min with Nb-IFN in RPMI 5% fetal calf serum at 37 °C and then labelled with anti-phospho-STAT1 and anti-PD-L2 antibodies. FACS data were acquired using a BD FACS Canto and analysed using either Diva (BD Biosciences) or FlowJo (TreeStar) softwares. How to cite this article: Garcin, G. et al . High efficiency cell-specific targeting of cytokine activity. Nat. Commun. 5:3016 doi: 10.1038/ncomms4016 (2014).